Sight of parasitoid wasps accelerates sexual behavior and upregulates a micropeptide gene inDrosophila Parasitoid wasps inflict widespread death upon the insect world. Hundreds of thousands of parasitoid wasp species kill a vast range of insect species. Insects have evolved defensive responses to the threat of wasps, some cellular and some behavioral. Here we find an unexpected response of adult Drosophila to the presence of certain parasitoid wasps: accelerated mating behavior. Flies exposed to certain wasp species begin mating more quickly. The effect is mediated via changes in the behavior of the female fly and depends on visual perception. The sight of wasps induces the dramatic upregulation in the fly nervous system of a gene that encodes a 41-amino acid micropeptide. Mutational analysis reveals that the gene is essential to the behavioral response of the fly. Our work provides a foundation for further exploration of how the activation of visual circuits by the sight of a wasp alters both sexual behavior and gene expression. Drosophila in the wild suffers massive mortality from the attacks of parasitoid wasps. As many as 80% of Drosophila larvae in natural environments may be killed by wasps that lay eggs in them [1] . These eggs hatch into larval wasps that devour the fly larva from within [2] . Adult wasps then emerge and mate, after which female wasps search for new hosts in which to begin the cycle anew [3] . As many as 350,000 species of parasitoid wasps may inhabit the natural world [4] , an indication of their enormous importance in ecology and evolution. The species they parasitize have evolved diverse defenses to protect themselves against these parasitoids. Some defenses operate at the cellular level. Attacked larvae, including those of Drosophila , may encapsulate the wasp egg with hemocytes and melanin [5] . Other larval defenses act at the behavioral level. Drosophila larvae show a remarkable rolling response at the onset of a wasp attack [6] , [7] . The larva rolls toward the wasp, winding its ovipositor around the larval body. This rolling often flips the wasp off balance and ends the attack. Adult Drosophila behavior is also affected by exposure to wasps. Female flies reduce their rate of oviposition, which may allow the female to lay more eggs later at another oviposition site where the threat of wasp attack is lower [8] , [9] . Females exposed to wasps also prefer to lay eggs in food sources that contain alcohol, to which developing wasps may be more sensitive than developing flies [10] . These diverse defensive behaviors are driven by different kinds of neurons. Rolling behavior of larvae is mediated by nociceptive neurons [6] , and the reduction in oviposition can be driven by visual cues [8] , [10] . A dedicated olfactory circuit detects odors of parasitic wasps and drives aversion responses. In larvae, olfactory receptor Or49a detects the wasp odor iridomyrmecin and drives an avoidance response [11] . In adult flies, Or49a is coexpressed with Or85f, a receptor that detects the wasp odors actinidine and nepetalactol in a class of antennal neurons called ab10B [11] . These neurons drive avoidance of food substrates and oviposition sites that contain wasp odors. Along with the search for food sources and oviposition sites, mating is one of the most robust and essential of Drosophila behaviors. The mating behavior of fruit flies has been studied for over 100 years [12] . Males and females exchange a variety of cues, and successful mating depends on the execution of stereotyped male behaviors and on female receptivity [13] . Given the high frequency at which flies and their parasitoids encounter each other in nature, we wondered whether flies had evolved a mechanism that would allow mating behavior to respond adaptively to the presence of parasitoids. Here we find that exposure to parasitoid wasps affects sexual behavior between male and female flies: surprisingly, it is accelerated. Flies begin to copulate more quickly. The effect is observed in five different species of Drosophila , and can be induced by several species of parasitoid wasps that parasitize Drosophila , but not by species that do not. The effect depends on visual cues, is eliminated by a mutation ablating photoreceptor function, and is impaired in a fly in which LC4 visual projection neurons (VPNs) are blocked. Sexual behavior is affected after a female fly has been in visual contact with a wasp in a different compartment. This visual contact induces expression of a gene encoding a micropeptide of 41 amino acids in the Drosophila nervous system. Mutational analysis shows the gene is required for the mating acceleration. These results implicate a micropeptide in a novel behavioral response to a threat that is widespread in the insect world. We asked whether the mating of male and female fruit flies would be affected by the presence of parasitoid wasps. We placed a pair of D. melanogaster flies in a small Petri dish, either with or without parasitoid wasps (Fig. 1a ). In an initial experiment we used the wasp Leptopilina boulardi , which specializes on D. melanogaster and on closely related fly species [14] . Fig. 1: Exposure of Drosophila to wasps accelerates sexual behavior. a Courtship arena containing a male and virgin female fly with (left) and without (right) two wasps, one male and one female. b Copulation latency of D. melanogaster . p < 0.0001, two-tailed Mann–Whitney test, n = 105 for +Lb, i.e., exposed to wasps, n = 102 for unexposed, error bars = SEM. The experiment was allowed to run for 1 h. c Copulation latency of other Drosophila species while in arena. Four wasps, two males and two females, were used for exposure. Two-tailed Mann–Whitney test. D. simulans , p = 0.0035, n = 67 (exposed), n = 63 (unexposed); D. yakuba , p = 0.0001, n = 62, 63; D. biarmipes , p < 0.0001, n = 62, 62; D. willistoni , p = 0.0009, n = 93, 92. Error bars = SEM. d Competition paradigm. In the left vial, fluorescently labeled flies (green) are incubated with wasps; in the right vial, unlabeled flies are incubated without wasps; in the arena below, a labeled exposed fly and an unlabeled unexposed fly of the same sex are allowed to compete for a fly of the opposite sex. d ′ Competition paradigm. In the left vial, unlabeled flies are incubated with wasps; in the right vial, labeled flies are incubated without wasps; in the arena below, an unlabeled exposed fly and a labeled unexposed fly of the same sex are allowed to compete for a fly of the opposite sex. e Left, competition between a male exposed to L. boulardi and an unexposed male for an unexposed female; dark shading indicates the percentage of competitions won by the exposed male ( p = 0.843, chi-squared test, n = 102). Right, a female exposed to L. boulardi and an unexposed female are placed in an arena with an unexposed male; dark shading indicates the percentage of pairings in which the exposed female copulated ( p = 0.0038, chi-squared test, n = 115). f Experiments comparing the mating success of an exposed and unexposed female of other species, placed with a male of the same species. Chi-squared test. D. simulans ( p = 0.0129, n = 102); D. yakuba ( p = 0.0350, n = 119); D. biarmipes ( p = 0.0001, n = 84); D. willistoni ( p = 0.0057, n = 119). Full size image We expected that the presence of the parasitoids, a lethal threat to reproductive success, would delay mating. We were surprised to find exactly the opposite. In the presence of the wasps, the mean time to copulation was 16 min, compared to 25 min in the absence of the wasp, i.e. a 36% reduction in copulation latency (Fig. 1b , **** p < 0.0001, two-tailed Mann–Whitney test, n = 105, 102). The exposure to wasps did not reduce the fraction of pairs that copulated in this experiment: copulation occurred in 80% of pairs that were not exposed to wasps and in 86% that were exposed (p > 0.05, chi-squared test). We then tested four additional Drosophila species closely related to D. melanogaster and found the same acceleration to copulation in all four (Fig. 1c ). Exposure to wasps could affect the behavior of either the male fly or the female fly. We tested these possibilities through competition experiments. If exposure increased male motivation, we might expect an exposed male to outcompete an unexposed male when both males were placed in a chamber with a single unexposed female. We placed fluorescently labeled male flies in a chamber with wasps for 2 h, and in parallel placed unlabeled male flies in a separate chamber without wasps (Fig. 1d ). We then allowed a fluorescent exposed male to compete with an unexposed male for the same female in a small arena. To control for any effect of the fluorescent label, we also performed the reciprocal experiment, i.e. we exposed unlabeled males to wasps and allowed them to compete with unexposed, labeled males (Fig. 1d ′). The results of the two reciprocal experiments were scored blind and averaged. We found that exposed males and unexposed males were equally successful in mating competitions (Fig. 1e , left). By contrast, when we placed an exposed female and an unexposed female together with an unexposed male, in 63% of tests the exposed female was the one that copulated (Fig. 1e , right; ** p < 0.01, chi-squared test, n = 102, 115). These results suggested the hypothesis that exposure of females to wasps increases their receptivity to males. We tested this hypothesis by pre-exposing females of the other four Drosophila species to wasps. In all four cases, pre-exposed females were more likely to mate than non-exposed females (Fig. 1f ). We next asked whether exposure to other species of parasitoid wasps also accelerated mating behavior. We first tested Leptopilina heterotoma , which is closely related to L. boulardi , and subsequently Trichopria drosophilae and Asobara tabida ; all of these species have been shown previously to attack Drosophila melanogaster larvae or pupae [15] . When wasps of any of these three species were placed in an arena with a pair of D. melanogaster flies, copulation began sooner (Fig. 2a–c ). As a further test, a female fly that was pre-exposed to each wasp species was more likely to copulate than a non-exposed female fly when both were placed in an arena with a male (Fig. 2d–f ). Fig. 2: Effect of exposure to other insect species on sexual behavior of D. melanogaster . a Leptopilina heterotoma , n = 121 (exposed), 100 (unexposed). p = 0.0044, two-tailed Mann–Whitney test. Error bars = SEM. b Trichopria drosophilae , n = 67 (exposed), 67 (unexposed). p < 0.0001. c Asobara tabida , n = 81 (exposed), 85 (unexposed), p = 0.0051. g Drosophila suzukii , n = 121 (exposed), 119 (unexposed), p = 0.9592. h Muscidiflurax zaraptor , n = 101 (exposed), 101 (unexposed), p = 0.9568. Error bars in b , c , g , h are SEM. The statistical test used in b , c , g , h is a two-tailed Mann–Whitney test. In each case a male D. melanogaster and a virgin female D. melanogaster were placed in an arena with one male and one female of the indicated species. d – f , i , j A female D. melanogaster exposed to the indicated species and an unexposed female D. melanogaster were both placed in an arena with a male D. melanogaster as in Fig. 1d, d′ . Dark shading indicates the percentage of cases in which the exposed female mated. d L. heterotoma p = 0.0352, chi-squared test, n = 100. e T. drosophilae p = 0.0018, n = 100. f A. tabida p = 0.0464, n = 91. i D. suzuk ii p = 0.9196, n = 98. j M. zaraptor p = 0.5546, n = 103. The statistical test used in e , f , i , j is a chi-squared test. Full size image Does the presence of any other insects whatsoever accelerate Drosophila mating? The presence of another species of Drosophila, D. suzukii [16] , did not have any of these effects on the mating of a pair of D. melanogaster , and neither did the presence of Muscidiflurax zaraptor [17] , a parasitoid that deposits eggs in larger flies (Fig. 2g–j ). We hypothesized that the wasps that affected mating produced an odor that was not emitted by the other tested species, and that this odor activated a circuit that accelerated sexual behavior. Such an odor might be detected by Or49a, Or85f, or perhaps another receptor of the Or family [18] . If an Or were essential to the acceleration in copulation onset, then the copulation latency of flies mutant for the obligate Or co-receptor Orco [19] would be expected to be unaffected by exposure to wasps. However, we found that Orco mutant flies showed an acceleration in mating onset comparable to that of control flies following exposure to L. boulardi; the copulation latency was reduced by 38% (Fig. 3a ; compare to Fig. 1b ). Moreover, competition experiments again provided evidence of an effect on females but not males, as in control flies (Fig. 3b ). Similar results were obtained when L. heterotoma was used as the wasp (Supplementary Fig. 1a, b ). Fig. 3: Mating acceleration depends on visual cues. a Mating of an Orco 1 mutant is affected by exposure to L. boulardi . p = 0.0001, two-tailed Mann–Whitney test, n = 79 (exposed), 76 (unexposed). Error bars = SEM. b Left, competition experiments between an exposed Orco 1 male and an unexposed Orco 1 male, for an Orco 1 female ( p = 0.9042, chi-squared test, n = 69). Right, an exposed Orco 1 female and an unexposed Orco 1 female are placed in an arena with an Orco 1 male ( p = 0.0389, chi-squared test, n = 60). Dark shading indicates the percentage of cases in which the exposed animal mated. c An Ir8a; Orco 1 double mutant is affected by exposure to L. boulardi . n = 66 (exposed), 67 (unexposed), p = 0.0085. d Left, competition experiments between an exposed and unexposed IR8a; Orco 1 male, for an IR8a; Orco 1 female ( p = 0.8974, chi-squared test, n = 60). Right, an exposed and unexposed IR8a; Orco 1 female are placed in an arena with an IR8a; Orco 1 male ( p = 0.0223, chi-squared test, n = 62). e A nina B1 mutant is not affected by exposure to L. boulardi under room light, n = 67 (exposed), 66 (unexposed), p = 0.7904. We note that this mutant is slow to mate. f nina B1 is not affected by exposure to L. heterotoma under room light, n = 69 (exposed), 68 (unexposed), p = 0.9598. 2 male and 2 female wasps were used in e – j . g Our Canton-S wild type strain is not affected by exposure to L. boulardi under dim red light n = 74 (exposed), 74 (unexposed), p = 0.195. h Canton-S is not affected by exposure to L. heterotoma under dim red light n = 74 (exposed), 74 (unexposed), p = 0.6537. i Canton-S is affected by exposure to L. boulardi under green light, n = 68 (exposed), 68 (unexposed), p < 0.0001. j Our Canton - S wild-type strain is affected by exposure to L. heterotoma under green light, n = 64 (exposed), n = 65 (unexposed), p = 0.0005. k Exposure to L. boulardi affects copulation latency of parental control TNT: n = 63 (exposed), 63 (unexposed), p = 0.0001. l Exposure to L. boulardi affects copulation latency of parental control LC4: n = 82 (exposed), 79 (unexposed), p = 0.0076. m – p Flies in which LC4 neurons are blocked with TNT are not affected by exposure to the indicated four species of wasps: in m ( L. boulardi ), n = 84 (exposed), 78 (unexposed), p = 0.6211; in n ( L. heterotoma ), n = 80 (exposed), 78 (unexposed), p = 0.6289; in o ( Trichopria drosophilae ), n = 90 (exposed), 81 (unexposed), p = 0.4496; in p ( Asobara tabida) , n = 85 (exposed), 81 (unexposed), p = 0.643. Error bars in c , e – p are SEM. The statistical test used in c , e – p is a two-tailed Mann–Whitney test. Full size image Could the effect be mediated by an odor that activates an ionotropic receptor (IR) odor receptor [20] ? We tested flies doubly mutant for the Orco and IR8a co-receptors; IR8a is essential for many IR-mediated responses [21] . These double mutants again showed the same mating acceleration phenotypes, for both L. boulardi and L. heterotoma , and again pre-exposure of females but not males had an effect in competition experiments (Fig. 3c, d and Supplementary Fig. 1c, d ). Taken together, these results suggested that olfactory cues do not drive the acceleration of mating. We next tested the hypothesis that the mating effect depended on visual cues. Consistent with this hypothesis, we found that a visually impaired mutant that is defective in the synthesis of visual pigments, ninaB 1 (ref. [22] ), showed equivalent copulation latency in the presence and absence of L. boulardi (Fig. 3e ); the same result was found with L. heterotoma (Fig. 3f ). Likewise, when the assay was conducted in dim red light, to which Drosophila has very low sensitivity, copulation latency of wild type flies was not affected by the presence of either species of wasps (Fig. 3g, h ). As a control, we conducted the assay in green light (~500–565 nm), to which sensitivity is much higher, and we observed effects on mating (Fig. 3i, j ). The simplest interpretation of these results is that copulation dynamics is affected by visual cues emanating from wasps. Color cues are unlikely to be essential, however, since they should be minimal under green light. To test further the hypothesis that the effect of wasps on fly mating behavior is mediated by vision, we asked whether blockage of certain VPNs affected mating behavior. VPNs transmit information from the primary visual center of the brain, the optic lobe, to higher brain regions. The most numerous VPNs in the lobula are lobular columnar (LC) neurons, which fall into multiple types based on their anatomy [23] , [24] . Activation of different LC types with split-GAL4 lines evokes different behaviors [25] . Silencing of one class of LC neurons, LC4, has previously been shown to reduce the escape response of Drosophila to predators [26] , [27] . We used split-GAL4 lines to block LC4, and found that this blockage eliminated the effect of wasps on copulation latency. Parental control flies expressing a UAS-TNT transgene alone (“TNT”, Tetanus Toxin Light Chain , which cleaves synaptobrevin to block synaptic transmission), or split-GAL4 constructs alone (“LC4”), showed the expected reduction in copulation latency when exposed to L. boulardi (Fig. 3k, l ). However, flies in which LC4 neurons were blocked (“LC4, TNT”) did not show a reduction in copulation latency, when exposed to L. boulardi or any of three other tested species, L. heterotoma, Trichopria drosophilae or Asobara tabida (Fig. 3m–p ). Visual cues were found in an earlier study to drive the depression in oviposition that follows exposure of flies to wasps [28] . In that study, visual cues from wasps in one transparent chamber were shown to affect the behavior of flies in an adjacent chamber. We found that cues from wasps could also affect sexual behavior of flies that were in visual contact with them from another chamber; copulation latency was accelerated (Fig. 4a ). In this initial experiment male flies and female flies were exposed to wasps separately and then allowed to mate. We also found that female flies exposed in this manner showed accelerated copulation latency when allowed to mate with unexposed male flies (Fig. 4b ), consistent with our earlier findings that wasps affected female behavior (Fig. 1e, f ). Fig. 4: Sight of a wasp in another chamber affects sexual behavior of a fly. a Copulation latency of a male fly and a female fly that were each exposed separately to the sight of L. boulardi wasps for 2 h and then allowed to mate (+Lb, n = 83), compared to mating of an unexposed male and an unexposed female (−Lb, n = 82). p < 0.0001, two-tailed Mann–Whitney test. Error bars = SEM. b Mating of a female fly that was exposed to wasps and an unexposed male (+Lb, n = 71) compared to mating of unexposed flies (−Lb, n = 69), p = 0.0003. c Mating of a female fly that was exposed to female L. boulardi wasps exclusively, and an unexposed male fly (+Lb, n = 67) compared to mating of unexposed flies (−Lb, n = 67), p = 0.0094. d Mating of a female fly that was in visual contact with male L. boulardi wasps exclusively, and an unexposed male fly (+Lb, n = 63) compared to mating of unexposed flies (−Lb, n = 63), p = 0.0017. e Mating of a female fly that was in visual contact with female L. heterotoma wasps exclusively, and an unexposed male fly (+Lh, n = 65) compared to mating of unexposed flies (−Lh, n = 63), p < 0.0001. f Mating of a female fly that was exposed to male L. heterotoma wasps exclusively, and an unexposed male fly (+Lh n = 63) compared to mating of unexposed flies (−Lh, n = 62), p < 0.0001. g Mating of a female fly that was in visual contact with female T. drosophilae wasps exclusively, and an unexposed male fly (+Td, n = 63) compared to mating of unexposed flies (−Td, n = 62), p = 0.0058. h Mating of a female fly that was in visual contact with male T. drosophilae wasps exclusively, and an unexposed male fly (+Td, n = 67) compared to mating of unexposed flies (−Td, n = 65), p = 0.0014. i Mating of a female fly that had been in visual contact with wasps (male and female) for 2 h and then isolated for 2 h before pairing with a male fly ( n = 69) compared with mating of an unexposed female ( n = 69), p = 0.7669. j Mating of a female that had been in visual contact with wasps for 24 h and allowed to mate with an unexposed male ( n = 68) compared with mating of an unexposed female ( n = 68), p = 0.0038. Error bars in b – j are SEM. The statistical test used in b – j is a two-tailed Mann–Whitney test. Full size image Since only female wasps are a threat to flies, we hypothesized that only female wasps would affect the mating behavior of a female fly. Female L. boulardi have much shorter antennae than males. However, we found that visual contact with either female or male L. boulardi wasps affected copulation latency (Fig. 4c, d ). We also tested two other wasp species, L. heterotoma and Trichopria drosophilae , in which the antennae are also shorter in females than males, and found the same results (Fig. 4e–h ). Is the effect on the female flies permanent? We allowed female flies to be in visual contact with wasps for 2 h, and then kept them apart from wasps for 2 h before testing them with males. We found that the effect was not permanent: there was no difference between the mating behavior of exposed female flies that had been away from wasps for 2 h and unexposed female flies (Fig. 4i ). We hypothesized that if we increased the time of exposure by an order of magnitude, that female flies would adapt to the cues and their mating would no longer be affected. However, we found that if female flies were in visual contact with L. boulardi for 24 h and then tested, mating was accelerated. In fact, the copulation latency was reduced severely, by 46% (Fig. 4j ). We wondered if gene expression was affected by exposure to wasps in this paradigm. As an initial screen, we carried out a differential RNA-seq analysis of the heads of female flies that had been exposed to L. boulardi for 2 h and heads of unexposed females. We identified 10 genes whose expression level was increased significantly (adjusted p value < 0.05) in each of two differential expression platforms (Fig. 5a and Supplementary Fig. 2 ). Among these 10 genes, the one that showed the greatest increase was IBIN (Induced by Infection , a gene that encodes a micropeptide ) ; its expression increased by ~20× (the log 2 -fold change was 4.2 by CuffDiff and 4.6 by DESeq2). IBIN was not associated with a gene ontology (GO) term, but the other nine genes are associated with the GO terms “immune system” and/or “response to stress.” Six of these other genes encode canonical antimicrobial peptides. No gene showed a decrease in expression level by our statistical criteria. Fig. 5: Exposure to wasps affects gene expression. a Head transcriptomes of flies that have been in visual contact with L. boulardi for 2 h, and of control flies. The transcriptome is based on two biological replicates. FPKM fragments per kilobase of transcript per million mapped reads. b RT-qPCR analysis of IBIN . Exposure to L. boulardi or M. zaraptor was for 2 h. p = 0.046, 0.07, 0.0008, 0.019 (from left to right), ** p < 0.01, Mann–Whitney U test, two-tailed, n = 10. Error bars = SEM. c RT-PCR amplification from the indicated tissues. The eye tissue includes both retina and lamina. RT reverse transcriptase. The control gene is eIF3c . RT(−) refers to a negative control where no reverse transcriptase is added to ensure that genomic DNA is not being amplified. n = 2. d RT-qPCR analysis of IBIN from the indicated dissected tissues of flies that had been in visual contact with L. boulardi for 2 hv. from unexposed control flies. n = 3. Error bars = SEM. e RNA-seq reads ( y -axis = 0–8000 reads), n = 2. SignalP (version 5.0) was used to predict the presence of signaling peptide (SP in figure) and the cleavage site, and DeepLoc (version 1.0) was used to predict its extracellular localization. f Generation of a mutant IBIN 1 allele. Green indicates core promoter GAL4 sequences; red indicates 3XP 3-DsRed sequences. g , h Copulation latency of IBIN 1 mutant flies and wCS control flies that had been paired with wasps ( L. boulardi) . Two-tailed Mann–Whitney test, n = 67 in all cases. Error bars = SEM. In g , p < 0.0001 (left and right). In h , p = 0.377 (left), p = 0.1718 (right). Full size image We attempted to confirm and extend this result with quantitative real-time reverse transcriptase PCR (RT-qPCR). We again found an increase of ~20× in the expression of IBIN in the heads of females exposed for 2 h to L. boulardi relative to heads of unexposed females (Fig. 5b , left bar). Exposure to the parasitoid wasp M. zaraptor did not increase the level of IBIN (Fig. 5b ), just as exposure to this wasp did not affect mating behavior (Fig. 2h, j ). Blockage of LC4 neurons with UAS-TNT (“LC4 > TNT”) also eliminated the increase of IBIN induced by exposure to L. boulardi (Fig. 5b ), consistent with its inhibition of the behavioral effect (Fig. 3m ). As expected, parental control lines carrying UAS-TNT or split-GAL4 constructs alone showed increases following L. boulardi exposure, but not M. zaraptor exposure (Fig. 5b ). We confirmed these results in an independent experiment with different sources of tissue and a different method. We dissected eyes, optic lobes, and brain tissue from which optic lobes had been removed, and performed RT-PCR. An IBIN amplification product was easily visible in all three tissue preparations in flies that had been exposed to L. boulardi (Fig. 5c and Supplementary Fig. 3 ). The amplification product appeared upregulated compared to unexposed tissues in this initial PCR experiment. Upregulation of IBIN was not observed in LC4 > TNT flies (Supplementary Fig. 3 ). We then confirmed by RT-qPCR that IBIN was upregulated in all three of these tissues (Fig. 5d ; note log scale). The simplest interpretation of these results is that the micropeptide is upregulated in nervous tissue following exposure to L. boulardi . Remarkably, IBIN was recently shown to be induced in second-instar Drosophila larvae 48 h after infection by L. boulardi [29] . IBIN was also the gene most highly induced by infection of Drosophila adults with the bacterium Micrococcus luteus [29] . The gene is induced in immune-responsive tissues, and it can be activated by either the Toll or immune deficiency (Imd) pathways, which is unusual. Its overexpression leads to increased survival after bacterial infection, although the mechanism is unclear. Adult overexpression of IBIN also leads to elevation of sugar levels in the hemolymph, and of Hsp70Bb, a stress-responsive gene. An environmental stressor was also recently found to upregulate IBIN in males [29] . Four days of social isolation, a stressor that modulates behavior widely across animal phylogeny, upregulated IBIN in male heads. The IBIN gene was originally annotated as a long non-coding RNA and referred to as CR44404 or lincRNA-IBIN . However, it contains an open reading frame that is predicted to encode a micropeptide of 41 amino acids (Fig. 5e ). This micropeptide is conserved among a variety of Drosophila species (Supplementary Fig. 4 ). It is predicted to have a signal peptide that is cleaved so as to generate an extracellular micropeptide of ~23 amino acids. To test directly whether IBIN is required for the effect of wasp exposure on fly mating behavior, we generated a deletion mutation of IBIN by CRISPR/Cas9 genome editing (Fig. 5f ). We backcrossed the IBIN deletion allele for five generations against our control line to minimize the possibility of genetic background effects. We found that while the control line shows the expected acceleration in copulation latency with L. boulardi and L. heterotoma , the IBIN mutant did not (Fig. 5g, h ). The simplest interpretation of these results is that the micropeptide is required for the acceleration of mating behavior. We have found that the mating behavior of Drosophila accelerates following exposure to a parasitoid wasp. Exposed flies start mating more quickly. This acceleration effect is conserved among five Drosophila species tested, and the effect is elicited by exposure to several species of wasps that parasitize Drosophila , but not by other species that do not. We were surprised by the positive valence of the effect, i.e. an acceleration. In attempting to interpret this effect, we considered that parasitoid wasps are not a direct threat to adult flies, but rather to their offspring. Accordingly, if an opportunity to mate arises in the presence of a wasp, we speculate that it could still be beneficial to mate, but to complete the process expeditiously with a reduced investment of energy and time so as to conserve resources for the next, crucial step: the search for an oviposition site elsewhere with lower danger of wasp attack [30] . The effect is mediated by exposure of the female fly, as shown by the comparison of mating success between exposed and unexposed females (Fig. 1e ) and the finding that latency is shortened when females alone are exposed to wasps (e.g. Fig. 4b–g ). Perhaps females, which have greater parental investment than males in their offspring, have greater incentive to execute a mating strategy that improves the survival chances of their offspring. Thus the female fly would take advantage of the opportunity to mate, but would be influenced by the need to search for another food source for its offspring, a source where wasps are not present and a male fly may or may not be present. We note that both theory and experimental data support the existence of mechanisms by which exposure to parasitoid wasps may exert a rapid effect on aspects of fly reproduction (e.g. production of recombinant offspring [31] ); it is conceivable that the acceleration of mating we have observed is an aspect of such a mechanism. In interpreting this behavioral effect, it is important to appreciate the massive lethality imposed on Drosophila by parasitoid wasps in nature [1] . In an environment where 80% of larvae are killed by wasps, behavioral changes may be selected for strongly. The mating effects are mediated by vision, not olfaction, as demonstrated by their dependence on light, on a critical photoreceptor gene, and on visual system projection neurons that have previously been implicated in escape behavior [26] , [27] ; the role of vision is also consistent with the finding that fly mating is affected by visual contact with wasps held in a different chamber. The visual system also mediates the effects of wasp exposure on oviposition [10] , although the olfactory system mediates certain aversion responses in other paradigms [11] . The mating acceleration is elicited by exposure to several wasp species that parasitize Drosophila , but not by other species, inviting future investigation into the precise nature of the visual cues that drive this response. Visual contact with wasps is accompanied by changes in gene expression. A gene whose expression increases dramatically, IBIN , encodes a micropeptide of 41 amino acids. The increase in expression of this gene is reminiscent of the acceleration in mating, in the sense that it is elicited by wasps in a species-specific fashion and is dependent on the LC4 class of VPNs (Fig. 5b ). It is striking that the expression of this gene is also increased by two different stressors, social isolation [32] and immune challenge [29] . Following immune challenge, the gene is expressed in immune-responsive tissues, including hemocytes and the fat body. We found that after visual contact with wasps it is expressed in the nervous system: in eyes, optic lobe, and other brain tissue. The immune system and the nervous system share a variety of small signaling molecules, including neuropeptides that are produced by and that affect cells of both systems, such as neuropeptide Y [33] , [34] . There is also extensive communication between the two systems, with the function of each having an impact on the other. We note that two immune peptides, Diptericin B and GNBP-like 3, have recently been found to regulate long term but not short-term memory in Drosophila [35] . Further work will be required to determine whether the IBIN micropeptide represents a new link between the two systems. We have found via genetic analysis that IBIN is required for the mating acceleration that is induced by exposure to wasps. Our results now invite investigation of the secreted micropeptide that IBIN is predicted to encode. Micropeptides are being found to play roles in a rapidly expanding variety of processes in diverse animals and plants [36] . Further studies are needed to explore the possibility that it binds to a membrane-bound receptor, and to test the hypothesis that it is required for normal activity of neural circuits that control mating behavior. It will be of interest to determine, for example, whether the micropeptide affects the reduction in locomotor activity that is characteristic of female receptivity [37] , [38] . Taken together, our results extend the effect of parasitoid wasps to another domain of Drosophila behavior: mating. The presence of predators has been found to affect sexual behaviors in other species, including courtship, mate choice, and nest-building in fish [39] , [40] , [41] , calling behavior in tree frogs [42] , and mating behavior in birds [43] . We have examined the effect of exposure to parasitoids, an enormously abundant class of organism, and above all we have studied the effect in Drosophila , a species that allows incisive analysis of its underlying molecular, cellular, and circuit basis. Further analysis of the behavioral response we have found in Drosophila may have broad implications in the natural world. Flies We used our laboratory Canton-S (CS) stock of Drosophila melanogaster unless otherwise specified. Orco 1 had been backcrossed into a CS genetic background at least five times before using. The IR8a; Orco double mutant was from the laboratory of Richard Benton (Univ. Lausanne). Both Orco 1 and IR8a; Orco were validated via electrophysiology. nina 1 (also known as ninaB P315 ) was from the Bloomington Drosophila Stock Center. D. simulans, D. yakuba, D. biarmipes , and D.willistoni were from the Drosophila Species Stock Center. D. suzukii was from R. Cowles, Connecticut Agricultural Experiment Station. Additional ethics approval from a board is not required. LC4-SS00315 was from the Janelia Research Campus. UAS-TNT was outcrossed to our CS background at least five times before using. All flies were maintained on a standard cornmeal Drosophila medium (Archon Scientific Glucose Medium Recipe). Stocks were maintained at 22 °C in 50% relative humidity with a 12:12 light:dark cycle. For stocks maintained in vials, we kept a maximum of 20 females and 20 males together in a vial (9.5 cm height, 2 cm diameter, Archon Scientific) to prevent overcrowding. Stocks kept in bottles (9.5 cm height, 5 cm diameter at base, Archon Scientific) had a maximum of 80 females and 30 males. When flies were near eclosion, parents were removed from the bottles. Newly eclosed flies were transferred to fresh Drosophila media (bottles or vials at the same population density) and aged until between 3 and 8 days. Aging the flies on fresh media is important: flies aged on old media (i.e. the media in which they eclosed) appeared nutrient-deprived and laid few eggs. Parasitoid wasps Leptopilina boulardi (Lb17), Leptopilina heterotoma , Asobara tabida , and Trichopria drosophilae were kindly provided by Todd Schlenke (University of Arizona, Tucson AZ) [44] . In order to culture these wasps, adult Drosophila were allowed to lay eggs in vials containing standard Drosophila culture medium for 4 days before being replaced by adult wasps (10 females, 10 males), which then attacked the developing fly larvae. Wasps aged 3–7 days post-eclosion were used for all experiments. Fresh wasps were used for all experiments, such that wasps were never reused between experiments. Muscidifurax zaraptor was obtained from Rincon-Vitova Insectaries Inc. (Ventura, CA) as pupae and used after eclosion. Behavioral assays To test copulation behavior, a virgin male fly was paired with a virgin female fly, each 3–8-day-old, inside a 35 × 10 mm Petri dish containing Drosophila culture medium. The flies had been collected immediately after eclosion and housed in single-sex groups of 10–12 prior to the experiment. The Petri dishes already contained two male and two female wasps (exposed) or no wasps (unexposed), except that in Fig. 1b a single male wasp and a single female wasp were used. Flies and wasps were introduced into the Petri dish using an aspirator. Assays were conducted in a controlled behavioral room set to 25 °C, 50% relative humidity and in room light unless otherwise indicated. We measured copulation latency (time between the introduction of the male and female flies into the mating chamber and the initiation of copulation of each pair). The percentage of assays in which copulation occurred was not consistently greater for either exposed or unexposed flies. For competition experiments, we placed 10–12 virgin flies (males or females) in a Drosophila culture vial (9.5 cm height, 2 cm diameter) with 10 male and 10 female wasps for 2 h. Some flies were labeled, as indicated in some experiments, with UVXPBB UV fluorescent dye (maxmax.com), which had been applied to them by placing them in a vial with the dye and shaking gently, 2 days before the experiment began. We recorded the percentage of competitions won by the exposed fly. To minimize any effect of the label, we averaged the percentage won by the exposed fly in the case when it was fluorescently labeled with the percentage in the case when it was unlabeled; there was no obvious effect of the label. The experimenter did not know which fly was labeled until after the result had been scored. We estimate that copulation occurred in more than 95% of competition experiments, which were allowed to proceed for a maximum of 1 h. All statistical analysis used non-parametric tests. All experimental values were measured in parallel with age-matched controls. Within an experiment n values for experimental and control samples were comparable. We used a power analysis based on initial data (GPower 3.1 (ref. [45] )) to determine the minimum sample size for copulation latency experiments. Each replicate used different individual flies and wasps. Error bars = SEM. Exposure via visual contact In experiments in which female flies were allowed visual but not physical contact with wasps, 10–12 virgin females were placed in a vial (9.5 cm height, 2 cm diameter) with Drosophila culture medium, and the vial was surrounded by six equivalent vials containing culture medium with (exposed) or without (unexposed) 15 male and 15 female parasitic wasps for 2 h. Tissue preparation for RNA analysis Female flies were reared in parallel and kept at 22 °C, 50% humidity. For analysis of whole head RNA, within 1 min after exposure to wasps the flies were flash-frozen in liquid nitrogen and their heads were manually collected over dry ice. Ten heads of 7-day virgin females were collected in each replicate. For analysis of isolated head tissues, fly heads were submerged in phosphate-buffered saline and dissected with forceps under a stereomicroscope. In total, three biological replicates were prepared, each consisting of tissues pooled from five animals. RNA extraction For transcriptome analysis, RT-PCR, and RT-qPCR, tissues were ground in 300 µL RLT lysis buffer (Qiagen) and RNA was extracted by adding 300 µL acid phenol. Samples were heated to 65 °C for 10 min with interruption to vortex the samples. Residual phenol were removed from the aqueous phase with chloroform. Finally, the RNA was precipitated and then dissolved in water. A nanodrop was used to quantify the RNA. Transcriptome analysis RNA quality was determined by a bioanalyzer. RNA library preparation and Illumina HiSeq 2500 sequencing were carried out in the Yale Center for Genome Analysis. The RNA libraries were prepared according to the KAPA mRNA HyperPrep preparation procedure. ~30 million 75-nucleotide long paired-end reads were obtained and processed using the Tuxedo suite [46] . In short, reads were mapped to the Drosophila melanogaster genome (Dm6) with TopHat2, default settings, and were quantified used CuffDiff, default settings. In parallel, reads were counted using HTseq [47] and samples were compared using DESeq2, default settings [48] . Raw reads are accessible at the Genbank SRA database (BioProject accession number PRJNA642090). RT-qPCR cDNA was made from 1 µg of total RNA as a template using EpiScript according to the manufacturer’s protocol (Lucigen). qPCR was carried out with the iTaq Universal SYBR Green (Bio-Rad) system using ~100 ng of cDNA. Target gene expression was normalized to the level of EIF3c transcripts. 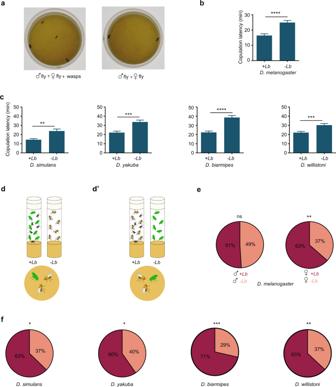Fig. 1: Exposure ofDrosophilato wasps accelerates sexual behavior. aCourtship arena containing a male and virgin female fly with (left) and without (right) two wasps, one male and one female.bCopulation latency ofD. melanogaster.p< 0.0001, two-tailed Mann–Whitney test,n= 105 for +Lb, i.e., exposed to wasps,n= 102 for unexposed, error bars = SEM. The experiment was allowed to run for 1 h.cCopulation latency of otherDrosophilaspecies while in arena. Four wasps, two males and two females, were used for exposure. Two-tailed Mann–Whitney test.D. simulans,p= 0.0035,n= 67 (exposed),n= 63 (unexposed);D. yakuba,p= 0.0001,n= 62, 63;D. biarmipes,p< 0.0001,n= 62, 62;D. willistoni,p= 0.0009,n= 93, 92. Error bars = SEM.dCompetition paradigm. In the left vial, fluorescently labeled flies (green) are incubated with wasps; in the right vial, unlabeled flies are incubated without wasps; in the arena below, a labeled exposed fly and an unlabeled unexposed fly of the same sex are allowed to compete for a fly of the opposite sex.d′ Competition paradigm. In the left vial, unlabeled flies are incubated with wasps; in the right vial, labeled flies are incubated without wasps; in the arena below, an unlabeled exposed fly and a labeled unexposed fly of the same sex are allowed to compete for a fly of the opposite sex.eLeft, competition between a male exposed toL. boulardiand an unexposed male for an unexposed female; dark shading indicates the percentage of competitions won by the exposed male (p= 0.843, chi-squared test,n= 102). Right, a female exposed toL. boulardiand an unexposed female are placed in an arena with an unexposed male; dark shading indicates the percentage of pairings in which the exposed female copulated (p= 0.0038, chi-squared test,n= 115).fExperiments comparing the mating success of an exposed and unexposed female of other species, placed with a male of the same species. Chi-squared test.D. simulans(p= 0.0129,n= 102);D. yakuba(p= 0.0350,n= 119);D. biarmipes(p= 0.0001,n= 84);D. willistoni(p= 0.0057,n= 119). 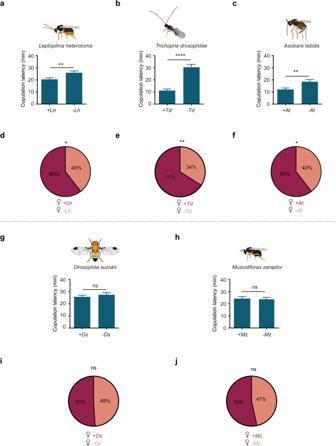Fig. 2: Effect of exposure to other insect species on sexual behavior ofD. melanogaster. aLeptopilina heterotoma,n= 121 (exposed), 100 (unexposed).p= 0.0044, two-tailed Mann–Whitney test. Error bars = SEM.bTrichopria drosophilae,n= 67 (exposed), 67 (unexposed).p< 0.0001.cAsobara tabida,n= 81 (exposed), 85 (unexposed),p= 0.0051.gDrosophila suzukii,n= 121 (exposed), 119 (unexposed),p= 0.9592.hMuscidiflurax zaraptor,n= 101 (exposed), 101 (unexposed),p= 0.9568. Error bars inb,c,g,hare SEM. The statistical test used inb,c,g,his a two-tailed Mann–Whitney test. In each case a maleD. melanogasterand a virgin femaleD. melanogasterwere placed in an arena with one male and one female of the indicated species.d–f,i,jA femaleD. melanogasterexposed to the indicated species and an unexposed femaleD. melanogasterwere both placed in an arena with a maleD. melanogasteras in Fig.1d, d′. Dark shading indicates the percentage of cases in which the exposed female mated.dL. heterotomap= 0.0352, chi-squared test,n= 100.eT. drosophilaep= 0.0018,n= 100.fA. tabidap= 0.0464,n= 91.iD. suzukiip= 0.9196,n= 98.jM. zaraptorp= 0.5546,n= 103. The statistical test used ine,f,i,jis a chi-squared test. Primers are provided in Supplementary Table 1 . Generation of an IBIN mutant A deletion was generated using CRISPR/Cas9 homologous recombination. The deletion lacks nucleotides 97–131 of the annotated IBIN transcript; it lacks most of the sequences encoding the predicted mature micropeptide and is predicted to create a frameshift mutation. Guide RNAs (gRNAs) were designed using the flyCRISPR Optimal Target Finder. gRNAs were cloned into pCFD4, a gift from Simon Bullock (Addgene # 49411) directly by PCR using Q5 polymerase (New England Biolabs), pCFD4 as a template. The PCR product, which contains both gRNA templates, was run on a gel and the resulting 600 bp band was gel-purified. In parallel, the original pCFD4 plasmid was digested with Bbs I and the linearized plasmid was also gel-purified. The gel-purified products were annealed by Gibson Assembly (NEB) according to the manufacturer’s instructions. The donor vector used for homology-directed repair was pHD-DsRed-attP, a gift from Melissa Harrison & Kate O’Connor-Giles and Jill Wildonger (Addgene #51019), with the Drosophila synthetic core promoter and Gal4 sequence from the pBPGUW plasmid, a gift from Gerald Rubin (Addgene #17575), cloned into the 5′ multicloning site, upstream of DsRed [49] . 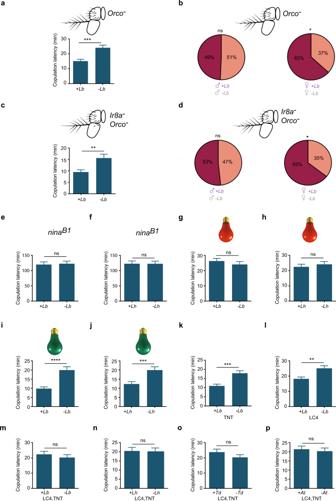Fig. 3: Mating acceleration depends on visual cues. aMating of anOrco1mutant is affected by exposure toL. boulardi.p= 0.0001, two-tailed Mann–Whitney test,n= 79 (exposed), 76 (unexposed). Error bars = SEM.bLeft, competition experiments between an exposedOrco1male and an unexposedOrco1male, for anOrco1female (p= 0.9042, chi-squared test,n= 69). Right, an exposedOrco1female and an unexposedOrco1female are placed in an arena with anOrco1male (p= 0.0389, chi-squared test,n= 60). Dark shading indicates the percentage of cases in which the exposed animal mated.cAnIr8a; Orco1double mutant is affected by exposure toL. boulardi.n= 66 (exposed), 67 (unexposed),p= 0.0085.dLeft, competition experiments between an exposed and unexposedIR8a; Orco1male, for anIR8a; Orco1female (p= 0.8974, chi-squared test,n= 60). Right, an exposed and unexposedIR8a; Orco1female are placed in an arena with anIR8a; Orco1male (p= 0.0223, chi-squared test,n= 62).eAninaB1mutant is not affected by exposure toL. boulardiunder room light,n= 67 (exposed), 66 (unexposed),p= 0.7904. We note that this mutant is slow to mate.fninaB1is not affected by exposure toL. heterotomaunder room light,n= 69 (exposed), 68 (unexposed),p= 0.9598. 2 male and 2 female wasps were used ine–j.gOur Canton-S wild type strain is not affected by exposure toL. boulardiunder dim red lightn= 74 (exposed), 74 (unexposed),p= 0.195.hCanton-S is not affected by exposure toL. heterotomaunder dim red lightn= 74 (exposed), 74 (unexposed),p= 0.6537.iCanton-S is affected by exposure toL. boulardiunder green light,n= 68 (exposed), 68 (unexposed),p< 0.0001.jOur Canton-S wild-type strain is affected by exposure toL. heterotomaunder green light,n= 64 (exposed),n= 65 (unexposed),p= 0.0005.kExposure toL. boulardiaffects copulation latency of parental control TNT:n= 63 (exposed), 63 (unexposed),p= 0.0001.lExposure toL. boulardiaffects copulation latency of parental control LC4:n= 82 (exposed), 79 (unexposed),p= 0.0076.m–pFlies in which LC4 neurons are blocked with TNT are not affected by exposure to the indicated four species of wasps: inm(L. boulardi),n= 84 (exposed), 78 (unexposed),p= 0.6211; inn(L. heterotoma),n= 80 (exposed), 78 (unexposed),p= 0.6289; ino(Trichopria drosophilae),n= 90 (exposed), 81 (unexposed),p= 0.4496; inp(Asobara tabida),n= 85 (exposed), 81 (unexposed),p= 0.643. Error bars inc,e–pare SEM. The statistical test used inc,e–pis a two-tailed Mann–Whitney test. In all, 1 kb length homology arms were PCR-amplified from Canton-S gDNA. Primers are provided in Supplementary Table 1 . 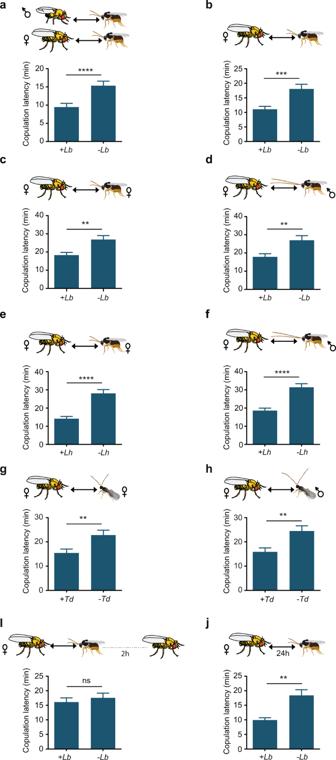Fig. 4: Sight of a wasp in another chamber affects sexual behavior of a fly. aCopulation latency of a male fly and a female fly that were each exposed separately to the sight ofL. boulardiwasps for 2 h and then allowed to mate (+Lb,n= 83), compared to mating of an unexposed male and an unexposed female (−Lb,n= 82).p< 0.0001, two-tailed Mann–Whitney test. Error bars = SEM.bMating of a female fly that was exposed to wasps and an unexposed male (+Lb,n= 71) compared to mating of unexposed flies (−Lb,n= 69),p= 0.0003.cMating of a female fly that was exposed to femaleL. boulardiwasps exclusively, and an unexposed male fly (+Lb,n= 67) compared to mating of unexposed flies (−Lb,n= 67),p= 0.0094.dMating of a female fly that was in visual contact with maleL. boulardiwasps exclusively, and an unexposed male fly (+Lb,n= 63) compared to mating of unexposed flies (−Lb,n= 63),p= 0.0017.eMating of a female fly that was in visual contact with femaleL. heterotomawasps exclusively, and an unexposed male fly (+Lh,n= 65) compared to mating of unexposed flies (−Lh,n= 63),p< 0.0001.fMating of a female fly that was exposed to maleL. heterotomawasps exclusively, and an unexposed male fly (+Lhn= 63) compared to mating of unexposed flies (−Lh,n= 62),p< 0.0001.gMating of a female fly that was in visual contact with femaleT. drosophilaewasps exclusively, and an unexposed male fly (+Td,n= 63) compared to mating of unexposed flies (−Td,n= 62),p= 0.0058.hMating of a female fly that was in visual contact with maleT. drosophilaewasps exclusively, and an unexposed male fly (+Td,n= 67) compared to mating of unexposed flies (−Td,n= 65),p= 0.0014.iMating of a female fly that had been in visual contact with wasps (male and female) for 2 h and then isolated for 2 h before pairing with a male fly (n= 69) compared with mating of an unexposed female (n= 69),p= 0.7669.jMating of a female that had been in visual contact with wasps for 24 h and allowed to mate with an unexposed male (n= 68) compared with mating of an unexposed female (n= 68),p= 0.0038. Error bars inb–jare SEM. The statistical test used inb–jis a two-tailed Mann–Whitney test. 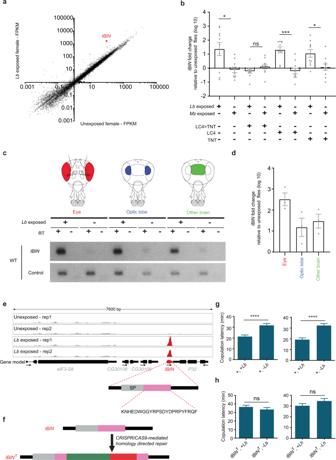Fig. 5: Exposure to wasps affects gene expression. aHead transcriptomes of flies that have been in visual contact withL. boulardifor 2 h, and of control flies. The transcriptome is based on two biological replicates. FPKM fragments per kilobase of transcript per million mapped reads.bRT-qPCR analysis ofIBIN. Exposure toL. boulardiorM. zaraptorwas for 2 h.p= 0.046, 0.07, 0.0008, 0.019 (from left to right), **p< 0.01, Mann–WhitneyUtest, two-tailed,n= 10. Error bars = SEM.cRT-PCR amplification from the indicated tissues. The eye tissue includes both retina and lamina. RT reverse transcriptase. The control gene iseIF3c. RT(−) refers to a negative control where no reverse transcriptase is added to ensure that genomic DNA is not being amplified.n= 2.dRT-qPCR analysis ofIBINfrom the indicated dissected tissues of flies that had been in visual contact withL. boulardifor 2 hv. from unexposed control flies.n= 3. Error bars = SEM.eRNA-seq reads (y-axis = 0–8000 reads),n= 2. SignalP (version 5.0) was used to predict the presence of signaling peptide (SP in figure) and the cleavage site, and DeepLoc (version 1.0) was used to predict its extracellular localization.fGeneration of a mutantIBIN1allele. Green indicates core promoter GAL4 sequences; red indicates 3XP 3-DsRed sequences.g,hCopulation latency ofIBIN1mutant flies andwCScontrol flies that had been paired with wasps (L. boulardi). Two-tailed Mann–Whitney test,n= 67 in all cases. Error bars = SEM. Ing,p< 0.0001 (left and right). Inh,p= 0.377 (left),p= 0.1718 (right). The homology arms were cloned into the modified pHD-DsRed-attP donor vector by Gibson Assembly. The finalized gRNA expression plasmid and donor vector were injected into embryos with germline-specific expression of Cas9 driven by the nanos promoter (y w; nos-Cas9(III-attP2)) by BestGene Inc. (Chino, CA). DsRed-positive alleles were then backcrossed to our control wCS line for five generations. Statistical analysis Statistical tests were performed in GraphPad prism (version 6.01). Reporting summary Further information on research design is available in the Nature Research Reporting Summary linked to this article.